Regioselective activation of benzocyclobutenones and dienamides lead to anti-Bredt bridged-ring systems by a [4+4] cycloaddition 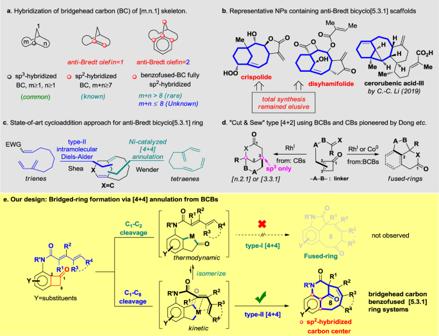Fig. 1: Representative natural products and design of a [4 + 4] annulation approach to access anti-Bredt bicyclo[5.3.1] skeleton. aHybridization of bridgehead carbon of [m.n.1] skeleton.bRepresentative NPs containing anti-Bredt bicyclo[5.3.1] scaffolds.cState-of-art cycloaddition approaches for anti-Bredt bicyclo[5.3.1] rings.d“Cut and sew” type [4 + 2] using BCBs and CBs pioneered by Dong, etc.eOur design: bridged ring formation via [4 + 4] annulation from BCBs. To the best of our knowledge, bridgehead carbon benzofused-bridged ring systems have previously not been accessible to the synthetic community. Here, we describe a formal type-II [4 + 4] cycloaddition approach that provides fully sp 2 -carbon embedded anti-Bredt bicyclo[5.3.1] skeletons through the Rh-catalyzed C 1 –C 8 activation of benzocyclobutenones (BCBs) and their coupling with pedant dienamides. Variously substituted dienamides have been coupled with BCBs to provide a range of complex bicyclo[5.3.1] scaffolds (>20 examples, up to 89% yield). The bridged rings were further converted to polyfused hydroquinoline-containing tetracycles via a serendipitously discovered transannular 1,5-hydride shift/Prins-like cyclization/Schmidt rearrangement cascade. Bridged ring systems are key structural motifs in many important functional molecules [1] , [2] , [3] . The skeleton were characterized by its size (e.g., bicyclo[m.n.1]) and ring strain (hybridization form of the bridgehead carbon (BC)). While the sp 3 -hybridized BC are commonly seen in many natural products, the sp 2 -hybridized BC underpins certain limitation on both the ring size (m + n ≥ 7) as well as ring strain [3] . However, consecutive sp 2 -hybridized carbon centers and/or bridgehead benzofused [m.n.1] systems are unusual (m + n > 8) and, to the best of our knowledge, unknown to chemist when it was confined in a small ring (m + n ≤ 8) framework (Fig. 1a ) [4] , [5] . We are herein set off to challenge these limitations. Bicyclo[5.3.1] bridged ring systems with anti-Bredt olefins at the bridgehead position are widely found in bioactive natural products (Fig. 1b ) [6] , [7] , [8] , whose total synthesis was highly dictated by the efficiency of assembling such scaffolds [9] , [10] . The state-of-art cycloaddition methods in constructing anti-Bredt bicyclo[5.3.1] scaffolds [11] , [12] , [13] , [14] are two: (1) type-II intramolecular Diels–Alder reactions developed by Shea et al. [15] , [16] , which requires activating substituent on dienophile, otherwise the reactions are mostly in gas phase; (2) a seminal report by Wender et al. [17] , [18] using Ni-catalyzed type-II [4 + 4] intramolecular cycloaddition under diluted conditions between 1,3-dienes (Fig. 1c ) [19] . A general, catalytic and diversifiable cycloaddition strategy remained elusive, especially for the highly strained anti-Bredt [20] , [21] bridged skeletons. The transition metal-catalyzed intramolecular [4 + 2] annulation via C 1 –C 2 bond activation [22] , [23] , [24] , [25] , [26] , [27] , [28] , [29] , [30] , [31] , [32] , [33] of benzocyclobutenones (BCBs) has emerged as an attractive approach for preparing fused- and bridged ring systems pioneered by Liebeskind [34] and Dong [35] , [36] (Fig. 1d ). However, no catalytic [4 + 4] annulation via oxidative C–C activation has been known, not to mention forming the highly strained anti-Bredt bridged ring systems [37] . Accessing anti-Bredt bridged bicycles remained elusive since only a few examples had been known starting from cyclobutanones [38] , [39] , [40] , [41] , [42] , [43] . To the best of our knowledge, no report had been known to construct bridged ring systems that bears highly strained consecutive double bond surrounding the BC. Fig. 1: Representative natural products and design of a [4 + 4] annulation approach to access anti-Bredt bicyclo[5.3.1] skeleton. a Hybridization of bridgehead carbon of [m.n.1] skeleton. b Representative NPs containing anti-Bredt bicyclo[5.3.1] scaffolds. c State-of-art cycloaddition approaches for anti-Bredt bicyclo[5.3.1] rings. d “Cut and sew” type [4 + 2] using BCBs and CBs pioneered by Dong, etc. e Our design: bridged ring formation via [4 + 4] annulation from BCBs. Full size image Herein, we disclose our discovery of a type-II [4 + 4] annulation between BCBs and dienamides enabled by Rh-catalyzed regioselective C 1 –C 8 bond activation (Fig. 1e ). The challenges are three-fold: (1) there is no precedent report of benzo-fused BC in bicyclo[5.3.1] systems; (2) the kinetically C 1 –C 8 rhodaindanone would be readily isomerize to its thermodynamically stable C 1 –C 2 cleaved counterpart [44] ; (3) competitive fused ring formation through normal cut and sew pathway. Our investigation commenced with preparation of 1a through amide formation in 72% yield between our previously reported 3-NHMe BCB and the known dienoic acid (see supporting information (SI) for detail) [45] . We tested our hypothesis by using 2.5 mol% of [Rh(nbd)Cl] 2 and 12 mol% of DPPP, unfortunately, only the fused tricycle 2a′ was isolated in 45% yield, presumably from the “cut and sew” process followed by a double bond migration (entry 1, Fig. 2 ). It is noted that the type-I [4 + 4] benzofused ring [46] , [47] product was not observed. When switching to other bidetate ligand with varied bite-angles, namely ( S )-H 8 -BINAP and ( S , S )-DIOP. Surprisingly, the desired anti-Bredt benzofused aza-bicyclo[5.3.1] bridged product 2a was successfully isolated (45% and 40% yield, respectively) together with the side product 2a′ (38% and 47% yield, respectively, entry 2 and 3). In both cases, product 2a ’s ee values were 0. These results led us to speculate that only one phosphine-center served as dative ligand based on the 18d-electron rule. Mono-dentate P(4-CF 3 Ph) 3 greatly improved the selectivity yielding only 2a in 51% yield (entry 4). However, the analogous P(C 6 F 5 ) 3 only lead to significantly decreased yield of 2a (21%) and selectivity (39% yield of 2a′ ), presumably due to the loose coordinating ability owing to its π-acidity as well as the large cone angle (entry 5) [48] . The electron-rich P(4-OMePh) 3 provided elevated yield (50%) of 2a albeit with 73% conversion (entry 6). Surprisingly, it was found that the feedstock PPh 3 provide the highest 72% isolated yield based on 85% conversion while preserving the complete selectivity for the bridged products (entry 7, with light yellow background). Encouraged by this result, a series of pre-catalysts were screened, but the yields of 2a ranged between 9 and 32% (entry 8–10). The Wilkinson catalyst was also used but proved less chemoselective as both 2a and 2a′ were obtained (entry 11). An attempt to lower the reaction temperature from 150 to 110 °C proved unfruitful, as 2a was only obtained in 10% yield with most of 1a recovered (entry 12). The Rh/ligand ratio was also proved crucial to the success of this [4 + 4] annulation pathway, since decreased efficiency (28% yield of 2a ) and loss of selectivity (38% yield of 3a ) was observed when lowering the loading of PPh 3 (entry 13). Toluene is an inferior solvent (entry 14). First row late transition metal are known to cleave C 1 –C 8 bond of BCB, but Co 0 and Ni 0 complex were tested and proved less efficient (entry 15–16). Fig. 2: Condition optimizations. Precatalysts, ligands, temperatures and their ratios have been screened. Full size image With optimal condition in hand, we set off to explore the reaction scope (Fig. 3 ). A broad series of dienamide coupled BCB substrates with different steric and electronic properties have been examined. Delightedly, good to high yields of bicyclo[5.3.1] bridged rings were obtained. It was found that changing the electronegativity of aryl substituents on δ-position of dienamides ( 1a–1d ) does not affect the efficacy, and 68–75% yields were obtained, with a slight trend for para -substituted effect favoring electron-withdrawing groups (entry 1–4, Fig. 3 ). The alkyl substituents at α and β-position of dienamide were also investigated (entry 5–8). It was gratifyingly to find that ethyl ( 1e ), cyclopropylmethyl ( 1f ) as well as hydrogen ( 1g–h ) at α-position were all well tolerated yielding desired bridged products 2e–h in useful yields (46–65%). It is noteworthy that no cleavage of cyclopropyl moiety was detected, revealing good chemoselectivity of this catalyst system. Variation of R group on the nitrogen promised potential use in complex settings, as 89% yield of 2i was isolated (95% brsm), when Bn ( 1i ) was used (entry 9). Increasing the steric bulkiness to cyclopropylmethyl ( 1j ) resulted in no less efficiency (79% yield of 2j , entry 10). The reaction demonstrated excellent chemoselectivity when 1k was employed as substrate, only bridged [4 + 4] product 2k (79% yield, 94% brsm) was observed but no traditional [4 + 2] product (entry 11). The robustness toward electronic variation on BCB was enlightened by obtaining 2l in 66% yield (81% brsm, entry 12). A grand challenge in “migratory insertion” is the unviability of sterically demanding multi-substituted olefins as coupling partners, presumably due to their low binding affinity. We postulated that dienamides are potential chelating ligands, which increased their binding ability to the rhodaindanone complex. The tetrasubstituted dienamide 1m was synthesized and the resulting [4 + 4] annulation product 2m (84% brsm yield) was undoubtedly verified through X-ray crystallography together with the aforementioned 2l (entry 12 and 13). A major competitive side reaction after migratory insertion is the tendency to undergo β-H elimination when a β-H is available. Gratifyingly, in our trials to effect the alkyl substituted dienamides 1n and 1o to the benzo-fused bridged skeletons, high to moderate yields were obtained, respectively, for 2n (89% yield) and 2o (52% yield) as the only isolated product in each case (entry 14 and 15). The terminal dienamide 1p underwent a certain decomposition which cause isolation of desired 2p in 31% yield albeit with moderate 67% brsm yield (entry 16). When the electronic property of dienamide was altered ( 1q ), the desired [4 + 4] annulation took place without loss of efficacy, obtaining 2q in 60% yield (entry 17). It was very encouraging to find that extended conjugated tetraenamide 1r react smoothly yielding 2r in 54% yield and the electron-rich furan moiety was well preserved (entry 18). When using even challenging (possessing cis -terminal olefins) cyclic dienamides 1s – u , the desired [4 + 4] annulation reactions proceeded without any difficulties, affording 2s ~ u in synthetically useful yields (54–58%, entry 19–21). The product 2t and 2u suggested that aromaticity can be deprived, since the X-ray crystallographic experiment undisputedly showed an exo -olefin for product 2u even with the possibility for re-aromatization (Fig. 3 , bottom). This might be caused by the highly strained anti-Bredt aza-bicyclo[5.3.1] skeleton. An effort to generate enantioselective bridged rings through chiral substrate induction was carried out using 1v , delightedly, the resulting product 2v and 2v′ was obtained in a 1:1 ratio as inseparable isomers in a combined 86% yield (entry 22). These provide valuable clues in our future endeavor toward enantioselective [4 + 4] annulation study. Additionally, we also found the ether substrate 1w yielded desired [4 + 4] product 2w , albeit in 12% yield. This indicated that our [4 + 4] conditions can be extrapolated to O linked diene substrate albeit in low yield (entry 23). Fig. 3: Substrate scope. 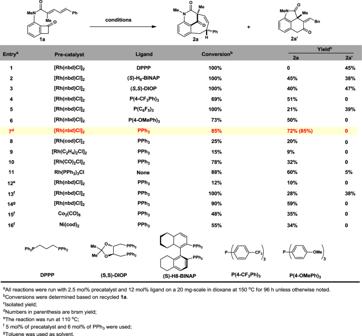Fig. 2: Condition optimizations. Precatalysts, ligands, temperatures and their ratios have been screened. a Conditions: all reactions were run with 2.5 mol% rhodium complex and 12 mol% ligand in dioxane at 150 °C for 96 h unless otherwise noted; b isolated yield; c numbers in parenthesis are brsm yields. X-ray structures were shown for compounds 2l , 2m , 2s , and 2u . Full size image With the highly diastereomerically pure benzo-fused bridged cyclic compounds 2 in hand, we hypothesized that if a Schmidt rearrangement reaction can be performed (Fig. 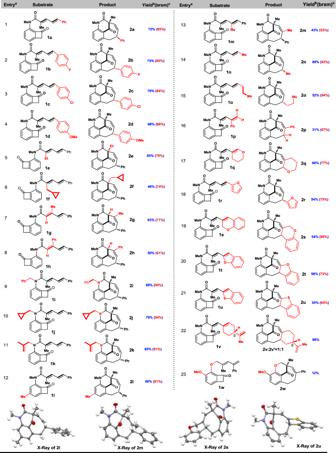Fig. 3: Substrate scope. aConditions: all reactions were run with 2.5 mol% rhodium complex and 12 mol% ligand in dioxane at 150 °C for 96 h unless otherwise noted;bisolated yield;cnumbers in parenthesis are brsm yields. X-ray structures were shown for compounds2l,2m,2s, and2u. 4 ), which would further extended the structural diversity [49] , [50] , [51] , [52] , [53] based on this [4 + 4] annulation strategy. In addition, it may be considered as a reaction surrogate for using the oxindole 3 as the annulation substrate, which has been an elusive substrate in C–C bond activation due to the more reactive amide bonds. Fig. 4: Derivatization hypothesis. We postulated that a Schmidt reaction of 2 maybe able to afford [5.3.2]bridged compound like 4 , which is very challenging using conventional C–C activation method. 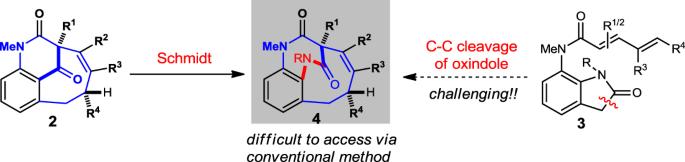Fig. 4: Derivatization hypothesis. We postulated that a Schmidt reaction of2maybe able to afford [5.3.2]bridged compound like4, which is very challenging using conventional C–C activation method. Full size image After extensive investigations, we were delighted to discover that the bicyclo[5.3.1] bridged tricycles can readily undergo a clean rearrangement reaction with isolated yields ranging from 51 to 62% yield (Fig. 5 ). A careful cultivation of a single crystal of the product 5g/5n and X-ray crystallographic analysis revealed that a densely functionalized and polyfused ring systems were obtained. Product 5 consists of a highly congested tetracyclic fused ring cycle rather than the designed simple Schmidt reaction in scheme 1. The mechanism of this transformation was probed using deuterated product 2a-D as substrate, which was synthesized from correspond 1a-D in 78% isolated yield using our standard [4 + 4] conditions (see SI for detail). The fused tetracyclic product 5a-D was successfully obtained in 64% yield indicating an unambiguous transannular 1,5-deuteryde transfer involved in the cascade skeleton rearrangement (Fig. 6 ). The dihydroquinoline moiety is a strong evidence of a cation-induced Schmidt rearrangement with NaN 3 presumably after the hydride shift (detailed mechanism is provided vide infra). Fig. 5: Cascade rearrangement for fuse-ring system. Conditions: 2 (1.0 equiv.) and H 2 SO 4 (5 drops) in TFA at 0 °C, then NaN 3 (3.0 equiv) at rt. X-ray structures was obtained for 5g and 5n + MeOH. Full size image Fig. 6: Mechanism probing of the cascade rearrangement. Standard conditions of [4 + 4] converted 1a-D to product 2a-D diastereoslelctively and with >95% Deuterium preserved. Standard conditions of cascade rearrangement afforded 5a-D with >95% Deuterium. Full size image Based on the previous report and the deuterium experiment, we tentatively proposed the catalytic cycle of the Rh-catalyzed [4 + 4] annulation between BCBs and pedant dienamides, together with the mechanism of the cascade skeleton rearrangement to form fused tetracycles from bridged bicyclo[5.3.1]undecane (Fig. 7 , upper cycle). The C 1 –C 8 oxidative addition with Rh I complex took place first regioselectively, and the equilibration from II to the C 1 –C 2 cleaved rhodaindanone (green) was competitively overrode by the regioselective migratory insertion into γ,δ-olefin due presumably to readily coordination with Rh-center. The resulting penta/hexa coordinated intermediate II was proposed to undergo a migratory insertion with the dienamide, yielding intermediate III . The Rh III complex III will undergo reductive elimination thanks to the excess PPh 3 ligand, providing the benzofused aza-bicyclo[5.3.1]undecandienone 2 . Fig. 7: Proposed mechanism. The upper catalytic cycle is the proposed mechanism for Rh-catalyzed type-II [4 + 4] cycloaddition, while the lower is the proposed mechanism for acid-catalyzed cascade rearrangement. Full size image To gain insight for our hypothesis of alkyl C 8 -Rh undergoing migratory insertion rather than acyl C 1 -Rh into the distal olefin, compound 6 was designed, prepared, and subjected to the standard [4 + 4] conditions. A formal [4 + 2 − 1] annulated product 7 was obtained in 76% yield (Fig. 8 ). The formation of product 7 indicated that C 8 -Rh migratory inserted into the terminal olefins first, followed by decarbonylation and reductive elimination. Otherwise, the decarbonylation could not be realized if acyl C 1 -Rh migrated first. Fig. 8: Control experiments. Substrate 6 was used to probe the mechanism of the migratory insertion step. Full size image In the cascade reaction (Fig. 7 , lower cycle), the bridged carbonyl group activated by catalytic H 2 SO 4 will initiated a through space 1,5-hydride transfer followed by a quick E1-type elimination from IV , affording hydride (pink) shifted intermediate V . The benzyl alcohol V will be protonated by the acid generating benzylic cation, which will induce a Prins-type cyclization obtaining VI . The intermediate VI will be trapped by NaN 3 and trigger a Schmidt rearrangement yielding the final polyfused hydroquinoline-containing tetracycle 5 . In summary, we have discovered a Rh-catalyzed type-II [4 + 4] annulation between BCBs and pedant dienamide constituting the first synthesis of the anti-Bredt bridgehead benzofused aza-bicyclo[5.3.1] ring system. 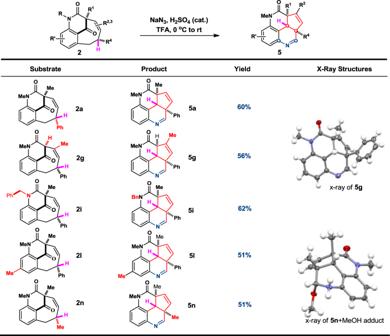Fig. 5: Cascade rearrangement for fuse-ring system. Conditions:2(1.0 equiv.) and H2SO4(5 drops) in TFA at 0 °C, then NaN3(3.0 equiv) at rt. X-ray structures was obtained for5gand5n+ MeOH. The methodology featured low catalyst loading (2.5 mol%) and neutral reaction condition with broad substrate scope (23 examples) and high efficiency (up to 89% yield). The mechanism probing experiment supported that an unusual alkyl C 8 -Rh bond undergoes migratory insertion into distal olefin first. To further diversify the anti-Bredt bridged ring systems, a cascade transformation consisting of transannular 1,5-hydride shift, E1 elimination, Prins-like cyclization, and Schmidt rearrangement was discovered, generating polyfused tetracyclic ring systems. 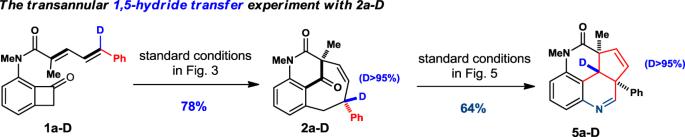Fig. 6: Mechanism probing of the cascade rearrangement. Standard conditions of [4 + 4] converted1a-Dto product2a-Ddiastereoslelctively and with >95% Deuterium preserved. Standard conditions of cascade rearrangement afforded5a-Dwith >95% Deuterium. A deuterated experiment supported the 1,5-hydride transfer mechanism. Procedure for rh-catalyzed type-II [4 + 4] annulation to make 2a A 4 ml oven-dried vial was transferred in a N 2 -filled glove box and was charged with 1a (40 mg, 0.126 mmol), [Rh(nbd) 2 Cl] 2 (1.5 mg, 3.15 μmol), PPh 3 (4.0 mg, 0.015 mmol), and 1,4-dioxane (3.7 ml) and the vial was capped. The vial was stirred at 150 °C for 96 h. Upon completion, it was cooled to room temperature. The solvent was removed by rotavap under reduced pressure and the residue was purified by flash chromatography to afford desired product 2a (28.8 mg) in 72% yield and partial 1a (4.9 mg) was recovered. The benzofused bicyclo[5.3.1] products can be further applied in a number of transformations (Fig. 9 ), Chemoselective reduction can be achieved by using different reagents, e.g., olefin could be hydrogenated obtaining saturated backbone 8 in 72% yield. Ketone and amide functional groups could be reduced to alcohol ( 9 in 82% yield as a single isomer) and methylene ( 10 in 60% yield), respectively, with different hydride reagents. In addition, product 2a could underwent nucleophilic attack with vinyl Grignard reagent yielding 11 as a single diastereoisomer (45% yield). When a methylene sulfur ylide was used, an expoxidation product will be isolated in 65% from 2l . A quasi-Favorskii reaction can be performed using aqueous NaOH, the fused tricycle product 13 was afforded in 30% yield. Fig. 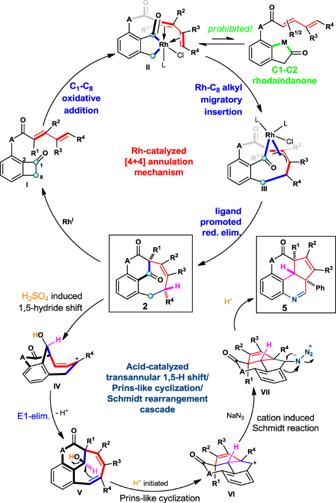Fig. 7: Proposed mechanism. The upper catalytic cycle is the proposed mechanism for Rh-catalyzed type-II [4 + 4] cycloaddition, while the lower is the proposed mechanism for acid-catalyzed cascade rearrangement. 9: Applications of compound 2. Hydrogentation with Pd/C afforded 8 . Selective reduction can be achieved chemoselectively obtaining 9 and 10 . 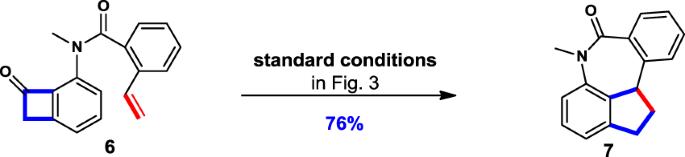Fig. 8: Control experiments. Substrate 6 was used to probe the mechanism of the migratory insertion step. 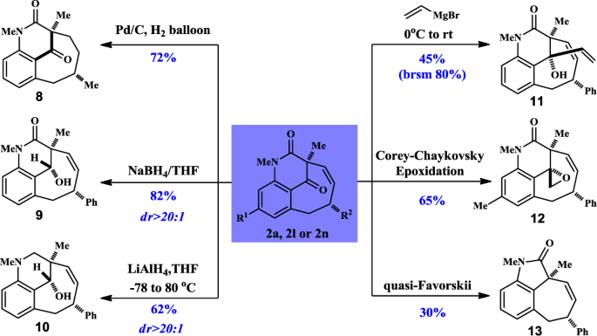Fig. 9: Applications of compound 2. Hydrogentation with Pd/C afforded8. Selective reduction can be achieved chemoselectively obtaining9and10. A 1,2-addition product11can be diastereoselectively obtained with vinylMgBr. Corey-Chaykovsky expoxidation provide12and quasi-Favorskii led to unexpected fused product13. A 1,2-addition product 11 can be diastereoselectively obtained with vinylMgBr. Corey-Chaykovsky expoxidation provide 12 and quasi-Favorskii led to unexpected fused product 13 . Full size image